Efficient organometal trihalide perovskite planar-heterojunction solar cells on flexible polymer substrates Organometal trihalide perovskite solar cells offer the promise of a low-cost easily manufacturable solar technology, compatible with large-scale low-temperature solution processing. Within 1 year of development, solar-to-electric power-conversion efficiencies have risen to over 15%, and further imminent improvements are expected. Here we show that this technology can be successfully made compatible with electron acceptor and donor materials generally used in organic photovoltaics. We demonstrate that a single thin film of the low-temperature solution-processed organometal trihalide perovskite absorber CH 3 NH 3 PbI 3-x Cl x , sandwiched between organic contacts can exhibit devices with power-conversion efficiency of up to 10% on glass substrates and over 6% on flexible polymer substrates. This work represents an important step forward, as it removes most barriers to adoption of the perovskite technology by the organic photovoltaic community, and can thus utilize the extensive existing knowledge of hybrid interfaces for further device improvements and flexible processing platforms. Photovoltaic uptake has been growing rapidly to make use of the world’s most abundant energy source, sunlight. Historically, conventional photovoltaics, namely crystalline silicon (c-Si), have been very expensive and this has led to a burgeoning field of research in solar technologies fabricated from fundamentally low-cost materials employing fundamentally low-cost fabrication methods [1] , [2] , [3] , [4] , [5] . Among these, the lowest cost and highest throughput method of fabrication is solution based reel-to-reel printing [6] . However, this has to be balanced with materials costs, other expenses such as environmental barrier protection and yield achievable when fabricating thin-film solar technologies at a high rate on flexible and deformable substrates. Over the last 5 years, there has been a continued downward drop in the price of c-Si solar cells to a level where the price of electricity from solar photovoltaics may have achieved grid parity in some parts of the world [7] . It is hence hard to envisage a solar technology breaking into the large-scale power market unless it can compete closely with c-Si on efficiency and then beat it on price. Thin-film solar cells, which are generally fabricated from vapour deposition of a solid semiconductor absorber film sandwiched between charge selective contacts, are slowly approaching the efficiencies of c-Si. However, the three most successful technologies, copper indium gallium (di) selenide, copper indium sulphide and cadmium telluride, all require deposition at relatively high temperature (~500 °C) and carefully controlled post deposition thermal treatments. This significantly limits the choice of possible substrates to those compatible with higher temperatures, and inhibits the possibilities of processing multiple cells on top of each other, required for high efficiency multi-junction device architectures. In contrast, organic photovoltaics can be processed very easily at low temperature, and has thus been able to capitalize upon the multi-junction approach to achieve efficiencies of over 10% [8] , [9] . However, in order to match c-Si on efficiency, organics still require at present a number of revolutionary step improvements in performance and device operation. Organometal trihalide perovskite absorbers are an appealing alternative photovoltaic technology, as they seem to combine the most appealing aspects of both thin film and organics: They can be processed under 150 °C, are fully solid-state and already exhibit high power-conversion efficiencies of between 12–15% when integrated into meso-superstructured solar cells (MSSC), [10] , [11] or perovskite-sensitized solar cells [12] , [13] . We have also very recently demonstrated their use in conventional vapor-deposited thin-film planar-heterojunction architectures, with over 15% efficiency [14] . Here, we demonstrate that the CH 3 NH 3 PbI 3-x Cl x perovskite absorber can be processed from solution, sandwiched between the conventional charge collection layers and electrode configuration for organic photovoltaic diodes. We demonstrate that a device structure consisting of fluorine-doped tin oxide (FTO)-coated glass, poly(3,4-ethylenedioxythiophene) poly(styrenesulphonate) (PEDOT:PSS), the perovskite absorber, [6,6]-phenyl-C 61 -butyric acid methyl (PCBM), TiO x and aluminium, (FTO/PEDOT:PSS/CH 3 NH 3 PbI 3−x Cl x /PCBM/TiO x /Al), as a planar heterojunction can deliver up to 10% power-conversion efficiency (PCE), and up to 6.5% for the same configuration on an indium-doped tin oxide (ITO)-coated plastic foil. This demonstrates the versatility of the perovskite absorber layer and indicates that the broader activities around organic photovoltaics can be applied towards the perovskite solar cell technology, greatly enhancing its potential to achieve over 20% efficiencies [15] and thus compete with the established c-Si industry. Furthermore, the structure developed in this work utilizes a p-contact to the FTO/glass substrate, thus leading towards the possible application of this technology in hybrid tandem solar cells, where the bottom cell is based on existing copper indium sulphide or c-Si technologies [16] . Device structure We have recently reported on perovskite-based thin-film photovoltaic devices with an architecture evolved from the solid-state dye-sensitized solar cells, where holes are collected through the metal cathode and electrons through the FTO anode [10] . In this configuration, a thin film of mesoporous alumina is deposited over compact TiO 2 -covered FTO substrates to aid the perovskite film formation [10] , then an organic hole transporter is deposited over the formed structure to provide a hole selective contact. Henceforth, this configuration will be referred to as ‘regular’ and the cell architecture, which represents the focus of the work here shall be termed ‘inverted’. Typical materials used in organic photovoltaics as hole selective contacts are PEDOT:PSS, V 2 O 5 and NiO [17] , [18] , while usually PCBM and more recently poly[(9,9-bis(3′-( N,N -dimethylamino)propyl)-2,7-fluorene)-alt-2,7-(9,9–dioctylfluorene)] (PFN) [19] are used as electron acceptors or electron selective contacts. In order to determine whether these materials are compatible to act as electron and hole acceptors within the perovskite-based devices, we first estimate photoluminescence (PL) quenching of the perovskite emission in thin-film bi-layers, as has become routine in all organic solar cells [20] . We present this data in Fig. 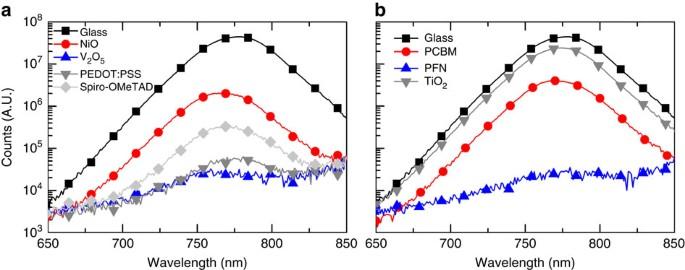Figure 1: Photoluminescence response for CH3NH3PbI3-xClxperovskite films coated withp- andn-type layers to ascertain their charge transfer compatibility. (a) Steady-state photoluminescence spectra ofp-type quenchers and (b)n-type quenchers of perovskite films processed in a bi-layer configuration. For thep-type quenchers, the perovskite was coated on top of thep-type collection layers, whereas for then-type quenchers, the perovskite was first processed on glass slides, then then-type charge collection layers were spin coated on top. Perovskite excitation at 530 nm was performed from the opposite side of the quencher. 1 and the results are summarized in Table 1 . All the p -type layers chosen in this work quench the perovskite steady-state PL more efficiently than the archetypal 2,2′,7,7′-Tetrakis[ N,N -di(4-methoxyphenyl)amino]-9,9′-spirobifluorene (spiro-OMeTAD) p -type hole conductor previously employed in the MSSCs, with similar values for PEDOT:PSS and V 2 O 5 of 99.8% quenching efficiency. All the n -type layers exhibit significantly higher quenching rates than the TiO 2 compact layers previously employed. Our observation of enhanced PL quenching with PCBM, is consistent with our previous work where we looked at electron transfer from the perovskite absorber to fullerene self-assembled monolayers, indicating that organic electron and hole acceptors are highly effective when interfaced with the perovskite absorbers [21] . All the cells fabricated in this work utilize a spin coated PCBM layer as the n -type contact, since solar cells fabricated with a PFN interlayer yielded an extremely poor photovoltaic performance. Figure 1: Photoluminescence response for CH 3 NH 3 PbI 3-x Cl x perovskite films coated with p - and n -type layers to ascertain their charge transfer compatibility. ( a ) Steady-state photoluminescence spectra of p -type quenchers and ( b ) n -type quenchers of perovskite films processed in a bi-layer configuration. For the p -type quenchers, the perovskite was coated on top of the p -type collection layers, whereas for the n -type quenchers, the perovskite was first processed on glass slides, then the n -type charge collection layers were spin coated on top. Perovskite excitation at 530 nm was performed from the opposite side of the quencher. Full size image Table 1 Steady-state photoluminescence quenching efficiency. Full size table When applied to devices, NiO and V 2 O 5 p -type layers resulted in rather poor photovoltaic performance ( Supplementary Fig. S1 ), showing signs of high series resistance and for V 2 O 5 a low shunt resistance in the J–V curves. This is likely to arise in part from extremely poor perovskite film formation upon the substrate, with very poor surface coverage ( Supplementary Fig. S2 ). This will enable direct contact of the PCBM n -type layer with the p -type metal oxide, presenting a shunting path. In addition, the high series resistance may arise from low conductivity of the p -type oxide, suggesting improvements could be made by controlling the conductivity or doping density in the p -type oxide, and improving the film formation of the perovskite upon the flat metal oxide layers. In contrast, when a thin PEDOT:PSS layer is used as the p -type contact, a solid perovskite absorber layer exhibiting over 95% surface coverage is achieved, as estimated from scanning electron microscopy (SEM) images, and the conductivity of the PEDOT:PSS is controlled and high. This results in good photovoltaic properties when a bi-layer of PCBM and compact TiO x is employed as the n -type charge collection layer. The origin of the different perovskite film formation characteristics on the different p -type layers is not completely understood at this moment and will be the subject of a future study, but is likely to originate from differences in surface roughness and perovskite/surface interaction energy [22] . To be able to process these structures in air, the top interlayer of TiO x was necessary to achieve a stable electronic contact with the top Al anode ( Supplementary Fig. S3 ) [23] . A cross-sectional SEM image of an optimized device is presented in Fig. 2 . 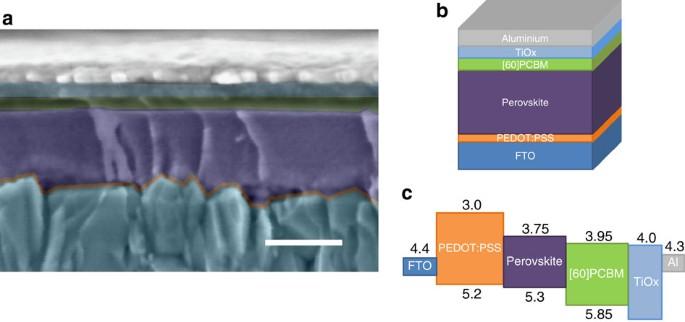Figure 2: Optimized device structure. (a) SEM. cross-sectional image of the optimized inverted device configuration. Scale bar represents 250 nm. The different layers have been tinted with the colour scheme of the device schematic shown in (b). (c) Approximate energy band diagram of the fabricated inverted structure taken from reference21. Figure 2: Optimized device structure. ( a ) SEM. cross-sectional image of the optimized inverted device configuration. Scale bar represents 250 nm. The different layers have been tinted with the colour scheme of the device schematic shown in ( b ). ( c ) Approximate energy band diagram of the fabricated inverted structure taken from reference [21] . Full size image Photovoltaic performance We show the photovoltaic performance of the inverted device structure in comparison with that of the regular MSSC device architecture (composed of a compact TiO 2 electron accepting layer, low temperature processed mesoporous alumina film filled with perovskite absorber and spiro-OMeTAD as the hole transporting layer) in Fig. 3 . The best performing device with the inverted architecture achieved a short-circuit photo current approaching 16 mA cm −2 , open-circuit voltages of over 0.9 V and 9.8% PCE, closely matching initial reports with devices based on the standard architecture. We also stress that this is achieved in a planar configuration, where no nanostructured scaffold is present and the total active layer thickness is around 300 nm. This good operation of the solid perovskite layer is consistent with our recent results where a planar heterojunction of a similar thickness composed of TiO 2 /CH 3 NH 3 PbI 3−x Cl x /Spiro-OMeTAD delivered over 15% PCE [14] . The PCE value shown here for inverted perovskite solar cells is higher than the best published single junction organic solar cells [19] , [24] , similar to the highest efficiencies for a-Si, and compares favourably with early reports of alternative thin-film technologies such as copper indium gallium (di) selenide, cadmium telluride [25] , with significant further improvements expected in the very near future [15] . A histogram for the PCE of a set of around 40 devices is also shown in Supplementary Fig. S4 as well as the photovoltaic performance of an inverted device under a series of light intensities from full AM 1.5 sunlight conditions to low <1% sunlight irradiation in Supplementary Fig. S5 . 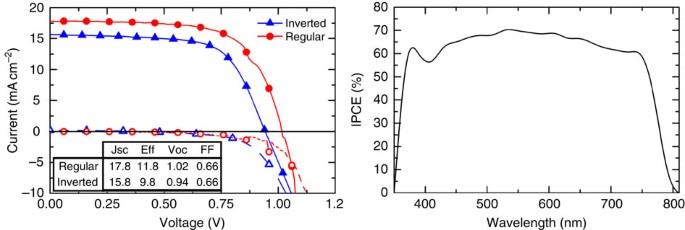Figure 3: Photovoltaic performance characteristics. (a) Current voltage curves for champion devices of regular MSSC (red circles) and inverted planar-heterojunction (blue triangles) configuration. Inset shows the short-circuit current density (Jsc, mA cm−2), power-conversion efficiency (Eff, %), open-circuit voltage (Voc, V) and FF for both device architectures. (b) Incident photon-to-electron conversion efficiency against wavelength for a typical inverted device. The integrated current from the product of the incident photon-to-electron conversion efficiency and the AM 1.5 100 mW cm−2solar spectrum is 16.5 mA cm−2, in close agreement to the short-circuit photocurrent measured under simulated sunlight. Figure 3: Photovoltaic performance characteristics. ( a ) Current voltage curves for champion devices of regular MSSC (red circles) and inverted planar-heterojunction (blue triangles) configuration. Inset shows the short-circuit current density ( J sc , mA cm −2 ), power-conversion efficiency (Eff, %), open-circuit voltage ( V oc , V) and FF for both device architectures. ( b ) Incident photon-to-electron conversion efficiency against wavelength for a typical inverted device. The integrated current from the product of the incident photon-to-electron conversion efficiency and the AM 1.5 100 mW cm −2 solar spectrum is 16.5 mA cm −2 , in close agreement to the short-circuit photocurrent measured under simulated sunlight. Full size image It is important to note that the J–V curves presented in this work were measured after aging the samples under constant light illumination for a number of minutes. The initial current voltage curve typically exhibit a little over >1% PCE, but increased to between 7.5–10% after around 10 minutes of constant illumination and operation in air ( Supplementary Fig. S6 ). This is not the case for the regular MSSC that operates well immediately. The requirement for light soaking of TiO x is consistent with previous reports in organic photovoltaics [26] . Flexible solar cells Finally, enabled by the ‘all low-temperature’ processing, we have also fabricated inverted perovskite devices on ITO-coated poly(ethylene terephthalate) (PET) substrates, shown in Fig. 4 . Devices fabricated on either ITO-covered glass or PET exhibited essentially the same photovoltaic performance parameters, with short-circuit currents of over 14 mA cm −2 , open-circuit voltages of around 0.9 V and power-conversion efficiencies of over 6.3%. The main difference between devices fabricated on ITO- and FTO-covered glass is the lower fill factor (FF) and current of the ITO devices. This may in part be accommodated by the batch–to-batch variation, but is likely to also arise from poorer perovskite film formation and lower surface coverage upon the PEDOT:PSS-coated ITO as opposed to the PEDOT:PSS-coated FTO, as shown in Supplementary Fig. S7 . The main difference between FTO and ITO is the surface roughness, with the latter being much smoother. It is likely that the roughness of the FTO is an important factor in enabling more uniform perovskite coating and ensuing better operation of these inverted perovskite solar cells, which do not incorporate any mesoporous scaffold. 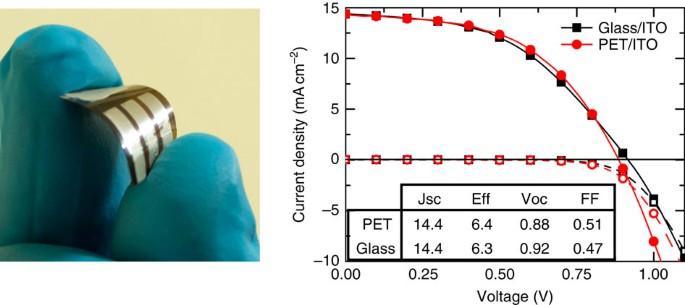Figure 4: Flexible solar cell performance. (a) Picture of the first flexible perovskite solar cell and (b)J–Vcurves for inverted architecture devices fabricated both on ITO-covered glass and PET, measured under-simulated AM 1.5 100 mW cm−2sunlight. The inset table shows the photovoltaic performance parameters,Jsc(mA cm−2), efficiency (%),Voc(V) and FF. Figure 4: Flexible solar cell performance. ( a ) Picture of the first flexible perovskite solar cell and ( b ) J–V curves for inverted architecture devices fabricated both on ITO-covered glass and PET, measured under-simulated AM 1.5 100 mW cm −2 sunlight. The inset table shows the photovoltaic performance parameters, J sc (mA cm −2 ), efficiency (%), V oc (V) and FF. Full size image The loss in PCE of 10% for the inverted devices as compared with 11.8% for the regular architecture arises from their slightly lower FF, short-circuit current and voltage. One of the key differences between our fabrication protocols for these two device architectures is that the compact TiO 2 layer is annealed to 500 °C in the regular MSSC. In order to check whether this could affect device performance, we have fabricated regular MSSCs with non-sintered compact TiO x layers. We observe the same requirement for light soaking as described in the photovoltaic performance subsection, and the same significant reduction in all photovoltaic performance parameters, especially FF ( Supplementary Fig. S8 ). This leads us to conclude that the presented inverted perovskite solar cell architecture should be capable of attaining the same efficiencies as the best performing MSSCs once a suitably effective TiO x or air stable n -type collection layer is employed. Another striking difference between the MSSCs and the presented inverted architecture is that in the former case, a mesoporous scaffold is used for the formation of the perovskite absorber, which presumably results in a structure where both perovskite and hole transporter are in close contact allowing efficient charge separation over short distances. In the inverted configuration presented here, a planar heterojunction is used. This implies that the majority of excitons or charges that are generated at/near the bottom of the device must travel the whole film thickness in order to be collected at the top contact. We have shown previously that this planar configuration also results in better performing solar cells when the perovskite film is deposited through a dual source vacuum deposition technique [14] , and is thus of a significant interest for future technology developments. In the optimization of the inverted solar cells, we fabricated devices with a range of perovskite thicknesses, from 100 nm up to 900 nm ( Supplementary Figs S9–S11 ). We obtained the best results with films of 300–400 nm, which absorb approximately 90% of the light that passes through the FTO-coated glass, integrated between 350–750 nm, taking into account the extended optical path length due to the presence of the Al ‘mirror’ as the top contact ( Supplementary Fig. S10 ). Devices fabricated from films of over 600 nm in thickness absorb more than 99% of the incident light; however, we found that the short-circuit currents for these thicker devices drop, and power-conversion efficiencies are maximized at around 400 nm thickness. As the exciton binding (E b ) energy is expected to be on the order of but slightly larger than the thermal energy (E b ~45 meV) ( [27] ), we expect a coexistence of excitons and free charge. At this stage, we do not know the branching ratio between free carriers and bound excitons, but this is an important factor to determine in order to understand the operating mechanism of these planar-heterojunction solar cells. The observed thickness dependence of the photocurrent sets a lower limit to the electron and hole diffusion lengths, whether they are excitons or free charge, of at least 400 nm in this mixed halide perovskite absorber. With the rapidly approaching commercial efficiencies and the tremendous versatility of the perovskite absorber demonstrated here, some concerns exist over potential toxicology issues of Pb in the current generations of organometal trihalide perovskites. However, thorough lifecycle analysis is required to correctly assess the scale of this issue, and the overall balance between the power generated from Pb-based PV and what pollution and toxic contamination is offset by such must be made. In addition, the perovskite-based solar cell technology is very young and a number of groups have already begun research to replace Pb with less toxic elements, which we can expect to lead to fruitful results in the near future [15] , [28] . In summary, organometallic perovskite solar cells offer the promise of a low-cost, mass-manufacturable solar technology that is compatible with current large-scale printing infrastructure. In this work, we have employed the ambipolar perovskite CH 3 NH 3 PbI 3−x Cl x , demonstrating fully air- and low-temperature processed solar cells exhibiting full sun power-conversion efficiencies approaching 10%. In doing so, we have demonstrated an ‘inverted’ architecture for perovskite-based photovoltaics where holes are efficiently collected from the FTO substrate through a PEDOT:PSS layer, and electrons from the top anode through a PCBM layer. We find that PEDOT:PSS functions as an excellent hole acceptor in this inverted system. The work presented here offers a new approach to design architecture for perovskite-based solar cells and is manufacturable on a broad range of substrates, including flexible plastic foils. In one sense, this demonstrates the versatility of the perovskite thin-film technology to the broad variety of possible device configurations, and equally importantly, this removes most barriers to adoption of the perovskite technology by the organic- and solution-processed photovoltaic community. Substrate preparation FTO-coated glass sheets (7 Ω/□ Pilkington) were etched with zinc powder and HCl (2 M) to obtain the required electrode pattern. The sheets were then washed with soap (2% Hellmanex in water), de-ionized water, acetone and methanol and finally treated under an oxygen plasma for 5 min to remove the last traces of organic residues. TiO x flat film precursor solution The TiO x flat film precursor solution consists of 0.23 M titanium isopropoxide (Sigma-Aldrich, 99.999%) and 0.013 M HCl solution in isopropanol (>99.9% Fisher Chemicals). To prepare this solution, titanium isopropoxide (369 μl) was diluted in isopropanol (2.53 ml) at 0.46 M. Separately, a 2 M HCl solution (35 μl) was diluted down with isopropanol (2.53 ml) to achieve a 0.026 M concentration. Finally, the acid-containing solution was added dropwise to the titanium precursor solution under heavy stirring. The solution was filtered with a PTFE filter with 0.2 μm pore size before use. Regular MSSC architecture fabrication The etched FTO substrates were coated with a compact layer of TiO 2 deposited by spin coating the TiO x flat film precursor solution at 2,000 r.p.m. for 60 s and consequently heating at 500 °C for 30 min. Then the mesostructured scaffold was deposited by spin coating a colloidal dispersion of ~20 nm Al 2 O 3 nanoparticles in isopropanol, followed by drying at 150 °C for 10 min. After cooling down to room temperature, the perovskite was deposited by spin coating from a DMF solution of methylammonium iodide and PbCl 2 (3:1 molar ratio), as described elsewhere [11] , which formed the perovskite after heating to 100 °C for 45 min in an oven. The hole transport layer was deposited by spin coating a 7 vol% spiro-OMeTAD solution in chlorobenzene with added 80 mM tert -butylpyridine and 25 mM lithium bis(trifluoromethanesulphonyl)imide at 1,000 r.p.m. for 45 s. Finally, devices were completed with evaporation in a high vacuum of Ag contact electrodes through a shadow mask. Inverted architecture fabrication The etched FTO substrates and ITO-covered glass and PET substrates were coated with a thin film of PEDOT:PSS deposited by spin coating a 25:75 vol% solution of PEDOT:PSS (Clevios):isopropanol (>99.9%, Fisher Chemicals), which was sonicated in an ultrasonic bath for 15 min and filtered with a 2.7 μm glass fibre filter before every use, at 2,000 r.p.m. for 60 s and subsequently annealed at 150 °C for 20 min (flexible substrates were mounted on a glass slide for spin coating). After cooling down, the perovskite precursor solution was spin coated at 2,000 r.p.m. for 20 s, and it was then heated to 100 °C for 45 min in an oven to form and crystallize the perovskite absorber. The electron selective contact was deposited by spin coating a 20 mg ml −1 solution of PC 60 BM in chlorobenzene (Anhydrous, Sigma-Aldrich) at 1,000 r.p.m. for 45 s. The TiO x flat film precursor solution was then spin coated at 3,000 r.p.m. for 45 s and the films were annealed at 130 °C for 10 min. Finally, devices were completed with evaporation in a high vacuum of Al contact electrodes through a shadow mask. NiO film deposition The spin coating precursor for the NiO thin film was prepared by dissolving nickel acetate tetrahydrate and monoethanolamine in ethanol, both at 0.1 M concentration under stirring in a sealed vial in air on a hotplate at 70°C for 4 h. The solution appeared homogenous and deep green. The solution was then spin coated at 2,000 r.p.m. for 45 s, directly on the FTO/glass substrate, and was further calcined at 500 °C for 45 min. V 2 O 5 film deposition The etched FTO substrates were coated with a thin film of V 2 O 5 deposited by spin coating a 1:35 vol% solution of vanadium (V)-oxytriisopropoxide (Sigma-Aldrich) in isopropanol and subsequently heated to 500°C to obtain crystalline vanadium oxide layers. The solution was then spin coated at 2,000 r.p.m. for 45 s, directly on the FTO/glass substrate, and was further calcined at 500 °C for 45 min. Measurement and characterization Solar-simulated AM 1.5 sunlight was generated with an ABET class AAB solar simulator calibrated to give 100 mW cm −2 using an NREL-calibrated KG5-filtered silicon reference cell. The spectral mismatch factor was calculated to be less than 1%. The J–V curves were recorded with a Keithley 2400. The active area of the solar cells was defined with a metal aperture mask of about 0.08 cm 2 . Steady-state PL measurements were taken using an automated spectrofluorometer (Fluorolog, Horiba Jobin-Yvon), with a 450 W xenon lamp excitation source and a photomultiplier tube detector. All spectra were corrected for instrumental response using a calibration lamp of known emissivity. SEM images were obtained using a Hitachi S-4300 microscope. How to cite this article: Docampo, P. et al. Efficient organometal trihalide perovskite planar-heterojunction solar cells for flexible polymer substrates. Nat. Commun. 4:2761 doi: 10.1038/ncomms3761 (2013).